Genomic adaptations of the halophilic Dead Sea filamentous fungusEurotium rubrum The Dead Sea is one of the most hypersaline habitats on Earth. The fungus Eurotium rubrum (Eurotiomycetes) is among the few species able to survive there. Here we highlight its adaptive strategies, based on genome analysis and transcriptome profiling. The 26.2 Mb genome of E. rubrum shows, for example, gains in gene families related to stress response and losses with regard to transport processes. Transcriptome analyses under different salt growth conditions revealed, among other things differentially expressed genes encoding ion and metabolite transporters. Our findings suggest that long-term adaptation to salinity requires cellular and metabolic responses that differ from short-term osmotic stress signalling. The transcriptional response indicates that halophilic E. rubrum actively counteracts the salinity stress. Many of its genes encode for proteins with a significantly higher proportion of acidic amino acid residues. This trait is characteristic of the halophilic prokaryotes as well, supporting the theory of convergent evolution under extreme hypersaline stress. The Dead Sea provides one of nature’s supreme tests of survival [1] . The negative-water balance of recent decades resulted in ever-rising salinity and divalent-cation ratios, cumulating in the current stasis. It’s brines reach a salinity level of 348 g l −1 total dissolved salts with a high ratio of Ca 2+ and Mg 2+ to Na + (ref. 2 ). Water activity (Aw, a measure based on the partial pressure of water vapour in a substance, and correlated with the ability to support microorganisms) of the Dead Sea is extremely low (Aw<0.669), even lower than that of saturated-NaCl solution (Aw=0.753±0.004) [3] , and is thus unbearable for most life forms. Nevertheless, a number of halobacteria (Archaea), one green algal species ( Dunaliella parva Lerche) [4] , and several fungal taxa withstand these extreme conditions [5] . Filamentous fungi from the Dead Sea are a focus of study since their discovery [6] . Essentially, most organisms in the Dead Sea survive in their dormant stages and only revive when salinity is temporarily reduced during rare heavy flooding events [7] or possibly by underwater fresh water springs [8] . In contrast, mycelial and spore stages of the ascomycete Eurotium rubrum W. Bremer are capable of surviving incubation in concentrated brines [9] . For counterbalancing environmental osmotic potentials in saline habitats, fungi synthesize or accumulate organic solutes, that is, osmolytes [10] , mainly glycerol, via the high-osmolarity glycerol (HOG) pathway [11] . This short-term response to increased salinity [12] has been investigated in great detail in the past few decades. In one experiment, a hog1 mutant of Saccharomyces cerevisiae (S. cerevisiae) , complemented by the EhHOG gene from a Dead Sea Eurotium strain, out-performed the wild type S. cerevisiae under lithium salt and freezing-thawing cycling [13] . However, these rapid and mostly transient responses are not considered responsible for long-term adaptation to high salinity [11] . To explain persistence of E. rubrum in one of the most extreme habitats on earth and understand its genomic and long-term functional adaptations, we sequenced the genome of this species and analyzed its transcriptomes during growth under hypo- and hypersalinity conditions. We show that the halophilic phenotype of E. rubrum is reflected in genomic modifications, such as specific gene gains and increased acidic amino acid content of proteins, highlighting various adaptive strategies of E. rubrum to the hypersaline-aquatic environment. Halotolerance of E. rubrum The strain E. rubrum CBS 135680 grew fastest at an Aw of 0.93 and ceases to grow without salts (Aw>0.97). Pure water has an Aw of 1.0, as Aw specifies the partial-vapour pressure of water in a sample divided by the standard state vapour pressure of pure water [3] . 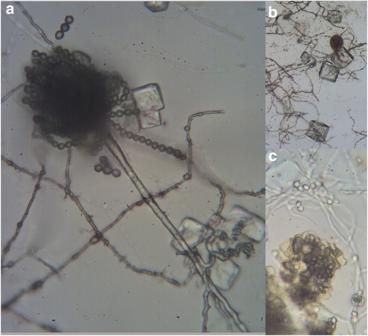Figure 1: Reproductive structures ofE. rubrumat high salt concentration. Strain CBS 135680, grown on sterilized glass slides in 60% DSW v/v liquid media. (a) Conidiophores and conidia (× 400); (b) Cleistothecia (× 100); (c) Asci and ascospores (× 400). Composition of the salts (that is, NaCl, MgCl 2 or diluted Dead Sea water (DSW), Supplementary Table 1 ) had no significant effect on growth rate and pattern ( Supplementary Fig. 1 ). Mycelial growth was maximal at 30% DSW (Aw~0.93) in both liquid and solid media ( Supplementary Fig. 1 ). E. rubrum regularly developed its characteristic reproductive structures [14] at salinities of 10–70% DSW. These included smooth hyaline conidiophores with radiating conidial heads forming ovate, finely roughened mitospores, e.g., conidia ( Fig. 1a ). Fruiting bodies, e.g., cleistothecia, were superficial, yellow to red brown, spherical and 80–120 μm in diameter ( Fig. 1b ). Asci were globose to subglobose, with eight ellipsoidal meiospores, e.g., ascospores ( Fig. 1c ). Malformation of the asexual-reproductive structures was observed under low-salt conditions ( Supplementary Fig. 2 ). Figure 1: Reproductive structures of E. rubrum at high salt concentration. Strain CBS 135680, grown on sterilized glass slides in 60% DSW v/v liquid media. ( a ) Conidiophores and conidia (× 400); ( b ) Cleistothecia (× 100); ( c ) Asci and ascospores (× 400). Full size image Phylogenetics of Eurotiomycetes Analyzing distances between ribosomal RNA gene internal-transcribed spacer sequences (ITS1) by non-metric multidimensional scaling revealed halotolerant strains in several distinct clusters of 4,197 Eurotialean sequences ( Supplementary Fig. 3 ). The phylogenetic reconstruction of 301 selected strains also showed a non-monophyletic origin of halotolerant strains ( Supplementary Fig. 4 ). A higher proportion of acidic residues in predicted proteins The 26.2 Mb genome of E. rubrum was sequenced, assembled and annotated to reveal 10,076 predicted genes with statistics resembling other sequenced Eurotiomycete genomes ( Supplementary Tables 2 and 3 ). The majority of E. rubrum proteins belong to gene families shared with nine other Trichocomaceae species ( Supplementary Table 4 ). Among the 10 strains, content of amino acids with aspartic and glutamic acid residues is highest in proteins of E. rubrum ( Supplementary Table 5 ), followed by the halotolerant Penicillium chrysogenum (Eurotiomycetes). The number of clusters with the highest content of acidic residues from E. rubrum was statistically significantly larger than expected by chance (Pearson’s χ 2 P <10 −4 ). By adding the two additional halophilic species Wallemia ichthyophaga [15] (Basidiomycota) and Hortaea werneckii [16] (Dothideomycetes), to the analyses, it became evident that gene families with high contents of acidic residues are particularly frequent in all three taxa ( Supplementary Tables 6 and 7 ). Comparative analysis of gene families The E. rubrum genome includes quite a number of gene families with significantly increased gene counts compared with other Eurotiomycete genomes ( Supplementary Table 8 ). Among these families are sugar-binding antiviral proteins (Pfam: PF08881), catalases (PF00199), stress responsive A-/B-barrel proteins (PF07876), two families encoding putative transposases (PF03184 and PF05699) as well as GIY-YIG endonucleases (PF01541) and Zn-finger proteins (PF00172). On the other hand, significant reductions are observed in gene families involved in primary and secondary metabolism (for example, hydrolases and beta-ketoacyl synthases) and metabolite transport (for example, sugar transporters) ( Supplementary Table 9 ). Gene families uniformly expanded or contracted in the three halophilic taxa E. rubrum , H. werneckii and W. ichthyophaga , were not detectable against nine other Trichocomaceae species, using clustering and Pfam domain analysis ( Supplementary Data 1 ). Independent annotation of transporter families in the three halophilic genomes revealed that although the total number of predicted transporters differs in three genomes according to the total proteome sizes, the share of transporters (~9%) is similar across all three genomes ( Supplementary Table 10 ). Some families, like H + or Na + F-type ATPases or P-types ATPases, are more abundant in H. werneckii and W. ichthyophaga relative to E. rubrum . On the other hand, more gene copies from families such as oligopeptide or K + transporters are found in E. rubrum . In the W. ichthyophaga genome, hydrophobins (cell wall proteins) comprise the most expanded gene family (23 genes). Furthermore, the corresponding proteins are enriched in acidic residues when compared with hydrophobins in other fungi [15] . However, E. rubrum has just one hydrophobin gene and H. werneckii completely lacks hydrophobins [16] . Microarray normalization and differential gene expression Four high-density, two-colour microarrays were used to analyze the transcriptome profiles of E. rubrum cultures grown at three different salt conditions: DSW diluted to 5, 30 and 50% (Aw~0.97, 0.93, 0.85) of its original concentration. We focused on transcriptional alterations between cultures grown at 5 and 30% DSW (low-to-medium salt comparison) and at 30 and 50% DSW (medium-to-high salt comparison), respectively ( Fig. 2 ). 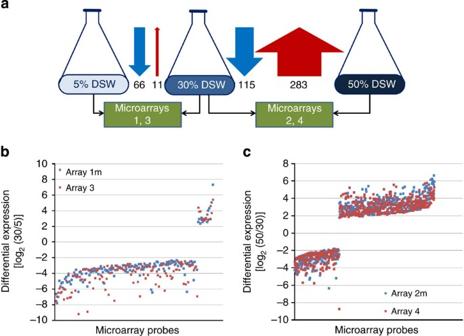Figure 2: Experimental overview and differential gene expression results inE. rubrumcultures grown at various salt conditions. (a) Labelled RNA transcripts from cultures grown in dilutions of DSW were combined and hybridized to four independent microarrays. The number of differentially expressed genes detected in replicate experiments, respectively, is depicted underneath the upward (induced in higher salt condition) and downward arrows (repressed in higher salt condition); arrow thicknesses are approximately to scale to the number of differentially expressed genes. Log-ratio distribution of induced (positive-log-ratio values) and repressed (negative-log-ratio values) genes in microarrays 1 m and 3 (b) and 2 m and 4 (c), respectively, identified by one-class differential expression analyses (microarray probes on horizontal axis in ascending order of the ‘statistics’ measure of the one-class analysis results; suffix ‘m’ indicates that the sign of the log-values were changed to account for dye-swap experiments). Figure 2: Experimental overview and differential gene expression results in E. rubrum cultures grown at various salt conditions. ( a ) Labelled RNA transcripts from cultures grown in dilutions of DSW were combined and hybridized to four independent microarrays. The number of differentially expressed genes detected in replicate experiments, respectively, is depicted underneath the upward (induced in higher salt condition) and downward arrows (repressed in higher salt condition); arrow thicknesses are approximately to scale to the number of differentially expressed genes. Log-ratio distribution of induced (positive-log-ratio values) and repressed (negative-log-ratio values) genes in microarrays 1 m and 3 ( b ) and 2 m and 4 ( c ), respectively, identified by one-class differential expression analyses (microarray probes on horizontal axis in ascending order of the ‘statistics’ measure of the one-class analysis results; suffix ‘m’ indicates that the sign of the log-values were changed to account for dye-swap experiments). Full size image Quality inspection, raw data normalization, and log-ratio transformation of the hybridization signals (Agilent feature extraction software) resulted in log-ratio values with the median close to 0.0, and an almost symmetric distribution of the 5 and 10 or the 90 and 95 percentiles, respectively ( Supplementary Fig. 5 ). However, the magnitudes of the ‘inner’ 25−50 and 50−75 percentile boxes were asymmetric among the four independent-microarray experiments, indicating a higher transcription rate of a considerable number of genes in cultures grown at 30% DSW compared with cultures grown at 5 and 50% DSW, respectively. This observation indicated an increased overall transcriptional activity on 30% DSW media, where cultures grew best. Additional normalization (within and between microarrays) was applied to the experiments using the Babelomics 4 gene expression suite [17] . The resulting box-plots of the normalized expression ratios showed similar log-ratio value distribution within and between the arrays ( Supplementary Fig. 5 ). Statistical analyses of the 5 versus 30% DSW microarray data sets using the LIMMA method (as implemented in Babelomics) revealed 14 microarray probes (11 genes) with significantly stronger hybridization signals, and 127 probes (66 genes) with significantly reduced hybridization signals at 30% DSW growth conditions ( Supplementary Data 2 ). A similar analysis using the 30 versus 50% DSW microarray data sets resulted in the identification of 340 microarray probes (283 genes) with increased- and 160 microarray probes (115 genes) with reduced-transcript levels at 50% DSW growth conditions ( Supplementary Data 3 ). GO enrichment analyses Analyses of gene ontology (GO) enrichment revealed that over the broad range of salinity from 5 to 30 to 50% DSW the transcript levels of several ion and solute transporters were significantly increased ( Table 1 ; Supplementary Data 2 and 3 ), with individual transporter genes specifically induced either at low- or high-salinity culture medium. In particular, metal ion transporters described as a CorA-like Mg 2+ transport protein, and a Fe 2+ /Zn 2+ -regulated transporter were elevated at medium rather than at low salinity. Other genes induced at medium-, but not at low-salt conditions, were an aspartic-type endopeptidase and a nicotinamide adenine dinucleotide phosphate-dependent quinone reductase ( Table 1 ; Supplementary Data 2 and 3 ). Compared with medium-salt concentrations, other metal ion transporters such as a putative zinc/iron permease, a voltage-dependent calcium channel, and a heavy-metal-transporting ATPase were upregulated at high salinity. In addition, members of the major facilitator superfamily many of them known as ‘secondary active solute transporters’ were only induced under high salinity. At high-salt conditions, gene products involved in beta-glucan biosynthetic processes and chitin binding were enriched. The glycerol-3-phosphate dehydrogenase is also significantly upregulated upon high-salt stress. Interestingly, genes induced only at high salinity also code for proteins assigned to cyclic AMP metabolic processes and to the regulation of cyclic nucleotide phosphodiesterases. Table 1 Gene Ontology (GO) term enrichment analyses. Full size table Among repressed genes at medium salinity compared with low salinity conditions (that is, ‘induced’ genes at low-salt conditions), the group of oxidoreductases (for example, the 3-hydroxy-isobutyrate and 4-hydroxy-phenlypyruvate dehydrogenases) and a series of transaminases were identified. The above-described significantly enriched-GO terms ( Supplementary Data 4 to 7 ) could be also visualized by GO graphs for the three major ontologies (biological process, cellular component and molecular function; Supplementary Figures 6 to 16 ). Fungi inhabiting hypersaline environments may either be halotolerant, growing at varying salt concentrations, or halophilic in the strict sense [18] , requiring a minimum concentration of salts for growth [19] . Halotolerance is widespread within Eurotiomycetes and aggregations of halotolerant strains into certain clusters in this analysis indicates genetic predisposition for this trait in various phylogenetic groups. Growth of the strain CBS 135680 at different salinities revealed that E. rubrum is a truly halophilic species. E. rubrum formed mitotic and meiotic reproductive structures, with viable spores in salt concentrations of up to 70% DSW (Aw~0.79), a dilution comparable with natural habitat conditions that caused a bloom in the Dead Sea in 1992 (ref. 20 ). In addition to the malformation of reproductive structures in low-salt conditions this observation clearly indicates the adaptation of the strain to hypersalinity. Accordingly, E. rubrum may be considered an active member of the microbial community in hypersaline environments [21] . A unique amino acid composition with large excess of acidic residues has already been recognized as a general trait of salt-adapted bacteria [22] , [23] . The genome of E. rubrum revealed that this applies to halophilic fungi, too, supporting the significance of high contents of acidic residues in proteins as an adaptation to saline environments [22] , [23] . Another mechanism of adaptation of organisms to low-water activities seems to be the adaptive duplication of specific genes. Highly xerotolerant strains of Zygosaccharomyces rouxii (Saccharomycetes) possess multiple copies of genes of the HOG pathway [24] , and evidence of duplications of genes involved in glycerol synthesis was reported from the genome of Xeromyces bisporus (Eurotiomycetes) [25] . H. werneckii kept duplicated genes involved in the regulation of fatty acid saturation [26] after its recent whole genome duplication [16] . While similar mechanisms were not observed for E. rubrum , other links to stress-response mechanisms were intriguing: significantly higher gene counts were observed for A-/B-barrel proteins, which are induced in salt-stressed plants [27] and for catalases, which remove reactive oxygen compounds accumulating under stress conditions. On the other hand, the halophilic fungi H. werneckii and W. ichthyophaga are enriched in genes encoding metal cation transporters [15] and P-type ATPase cation transporters [15] , respectively. Also, apparently hydrophobins are not obligatory for adaptation to high-salinity conditions. So, while halotolerance is obviously widespread within Eurotiomycetes and the aggregated occurrence of halotolerant strains in certain clusters indicate genetic predisposition for this trait in various phylogenetic groups, the differences in the gene content among the three examined halophilic fungal taxa suggest multiple molecular pathways for halo-adaptation and diversity in the mechanisms of halotolerance adopted by different fungi. Hardly any of the known short-term hypersalinity responses, for example, the HOG pathway [28] , cell wall integrity [29] , and ion homoeostasis via the Ca 2+ /calmodulin signalling pathway [30] were reflected by gene expression changes in E. rubrum under long-term hypo- and hypersaline stress. However, the glycerol-3-phosphate dehydrogenase, a key enzyme in the production of the compatible osmolyte glycerol [10] , is upregulated as in other halophilic fungi [31] . The study clearly indicated that long-term adaptation to salinity requires different cellular and metabolic processes than short-term osmotic stress signalling and perception. Transcription rates significantly increased at high salinity for genes related to ion and metabolite transport. Together with the observed loss of membrane transporter genes in comparison with other Eurotialean genomes, these findings reflect the need for tight control in transport of metabolites and ions across cell membranes under high salinity. Furthermore, the GO enrichment at high-salt conditions of gene products involved in beta-glucan biosynthetic processes and chitin binding indicated that the biophysical properties of the cell wall were adjusted under the high-salt environment. This clearly indicates that the fungus tries to cope ‘actively’ with its extreme environment and does not simply fall into dormancy, as might be expected by the greatly reduced growth rates. Understanding the long-term adaptation of cells and organisms to high salinity is of great importance in a world with increasing desertification and salination. The observed functional and structural adaptations provide new insight into the mechanisms that help organisms to survive under such extreme environmental conditions, but also point to new targets like the biotechnological improvement of salt tolerance in crops. Determination of halotolerance Halotolerance of E. rubrum strain CBS 135680 (KNAW-Fungal Biodiversity Centre) was tested at increasing salinity levels of 0–90% DSW. Corresponding levels were prepared using NaCl and 1:1 MgCl 2 :NaCl, respectively ( Supplementary Table 1 ). Spore suspensions (~10 2 ) prepared with 10% DSW, containing Tween 20 (0.05% final concentration), were spot inoculated in triplicate on Czapek-Dox broth (CzD, Sigma) plates containing corresponding salt concentrations. Growth was recorded in terms of colony diameter after 7 days incubation, or after 15 days for those showing no or delayed growth. In addition, growth of E. rubrum was tested in liquid CzD at corresponding salinities. One ml of spore suspension (~10 3 ) was inoculated into 100 ml of liquid media in 150 ml Erlenmeyer flasks and incubated on an orbital shaker (150 r.p.m.) at 27 ° C for 7 days. The mycelium was harvested, filtered, dried and weighed. To observe reproductive structures sterile glass slides were inserted into mature cultures of E. rubrum in liquid GY media (glucose 10 g l −1 , yeast extract 1 g l −1 ) using salt conditions as described (0–100% DSW) above and incubated for 1 week. Later, the slides were recovered and inspected using a light microscope for growth and formation of reproductive structures and spores, and photographed using a MD130 Electronic Eyepiece. Sequencing and assembly The E. rubrum genome and transcriptome were sequenced using the Illumina platform. For the genome, an unamplified whole genome shotgun library (250 bp insert) and one 4 kb long mate pair library were constructed, quantified by quantitative PCR, and sequenced on Illumina HiSeq 2000 in 2 × 100 bp reads format. Each fastq file was quality control filtered for artifact/process contamination and subsequently assembled with AllPathsLG release version R39750 (ref. 32 ). This resulted in a 26.2 Mb assembly in 110 scaffolds with 91.7 × read depth coverage ( Supplementary Table 2 ). The mitochondrial genome was assembled separately and resulted in a 39.7 × coverage assembly with one 51 Kb scaffold consisting of two contigs. Over 318 million RNASeq reads were obtained for the E. rubrum transcriptome and ab initio assembled into 30,179 contigs with a range of sizes between 100 and 17,830 bp (370 bp median). Of these, 92.49% were mapped to genome assembly with 95% identity and 80% coverage, which indicates a high level of completeness of the produced genome assembly. Genome annotation The E. rubrum assembly was annotated with the JGI annotation pipeline [33] , which combines multiple tools for gene prediction, annotation and analysis. Results were deposited in MycoCosm [34] ( http://jgi.doe.gov/fungi ) to allow further analysis and manual curation. The assembled genomic scaffolds were masked using RepeatMasker [35] with the RepBase 13.03 fngrep library of 234 fungal repeats [36] . Multiple tracks of gene models were predicted for each assembly, and automated filtering based on homology and EST support was applied to produce a final non-redundant GeneCatalog track representing the best gene model found at each genomic locus. The gene prediction methods were: transcriptome-based predictions with CombEST ( http://genome.jgi.doe.gov/programs/fungi/combest.jsf ) and ESTmap ( http://softberry.com ) using EST data comprising raw ESTs and assembled EST contigs; homology-based predictions with FGENESH+ (ref. 37 ) and Genewise [38] , with homology seeded by BLASTx alignments of the GenBank non-redundant sequence database (NR: http://www.ncbi.nlm.nih.gov/BLAST/ ) to the genomic scaffolds; and ab initio predictions using FGENESH pipeline [34] and GeneMark [39] . An additional GeneWisePlus track was generated by extending the 5′ and 3′ exons of GeneWise models to include 5′ start and/or 3′ stop codons when possible. Additional EST-extended tracks were generated using BLAST-aligned [40] EST contigs to add 5′ untranslated regions, 3′ untranslated regions, and Coding DNA Sequence (CDS) regions, supported by ESTs but omitted by the initial prediction methods. The non-redundant GeneCatalog model set produced from that assembly’s individual gene modeling tracks was subsequently subjected to further analysis and manual curation (see Supplementary Table 3 for gene model statistics). From the 10,076 gene models predicted in E. rubrum, 91% showed similarity to other proteins in NCBI non-redundant set (NR) and an absolute majority was supported by RNAseq data including 72% support over the entire gene length. All predicted gene models were functionally annotated by alignment similarity to annotated genes from the GenBank NR using BLASTp [41] and hardware-accelerated double-affine Smith-Waterman alignments (deCypherSW; http://www.timelogic.com/decypher_sw.html ) against SwissProt ( http://www.expasy.org/sprot )], the Kyoto Encyclopaedia of Genes and Genomes (KEGG) [42] , and eukaryotic orthologous groups of proteins (KOG) [43] ; analyzed for signal sequences and transmembrane domains with SignalP [44] and TMHMM [45] . Functional domains were predicted using InterProScan [46] . Enzyme commission EC numbers ( http://www.expasy.org/enzyme ) were assigned based on KEGG hits, and GO terms ( http://www.geneontology.org ) were assigned based on Interpro and SwissProt hits. Multi-gene families were predicted using the MCL Markov clustering programme [47] , based on pairwise BLASTp protein similarities. Using the 139,410 protein sequences of the 14 organisms in Supplementary Table 4 (with the exception of H. werneckii and W. ichthyophaga ) and an inflation parameter of 2 resulted in 36,910 clusters resulted with an average of 3.8 proteins per cluster. The majority of clusters (26,384) were singletons, suggesting the high degree of diversity in the proteins of the organism set used. Phylogeny inference A set of 221 clusters being single-copies in all organisms was identified and had the additional property that the BLAST alignment scores were sufficiently invariant (in an all-versus-all comparison, proteins with a minimum-score/maximum-score ratio <0.25 were excluded) in all sequences in every cluster. Using this set of 221 protein sequence clusters, protein sequences were concatenated and the MAFFT [48] programme was run with default options to generate a multiple alignment. The Gblocks programme [49] was then applied with options -t=p, -e=gb, -b4=5 to remove poorly aligned positions. Of the original 140,125 positions in the alignment, 89359 positions (63%) remained after Gblocks filtering. We used RaxML [50] to infer a phylogeny from the resulting filtered alignment of the 221 protein clusters. The PROTGAMMAWAG model was used, and Cryptococcus neoformans , Batrachochytrium dendrobatidis , S. cerevisiae , and Neurospora crassa were selected as outgroup taxa. Phylogenetics of Eurotiomycetes To obtain a representative set of Eurotiomycete sequences of the ITS1 NRDNA region from 506 well-referenced Eurotiomycetes, ITS sequences from earlier phylogenetic studies [51] , [52] were selected as a query seed. Sequences matching to one of these references with an e-value <1e−07 were downloaded from GenBank. The ITS1 region was extracted from 4,197 sequences found and the similarities were calculated and visualized by non-metric multidimensional scaling as described earlier [53] . The minimum-tolerated water activity was mapped to strains analyzed in this regard [3] . To infer phylogenetic relationships among the strains, the ITS sequences (ITS1, 5.8 S and ITS ribosomal RNA gene sequences) from earlier studies [51] , [52] were cleared from duplicates, that is, only one sequence was retained from identical sequences deposited under identical names. The remaining 267 sequences were aligned together with ITS sequences from strains experimentally tested for osmotolerance/halotolerance. The most likely phylogenetic tree was calculated from the unambiguously alignable positions using RAxML. CAFE analysis of gene families The CAFE programme [54] ( http://sites.bio.indiana.edu/~hahnlab/Software.html ) was used to analyze gains and losses in gene families in the 31 organisms. We used two methods of defining gene families for input to CAFE: assigning protein sequences to Pfam domains and assigning them to MCL [55] clusters. CAFE uses a stochastic model of gene death and birth to infer statistically significant gain and loss in gene families, given an ultrametric phylogenetic tree and a table of each organism’s number of copies of each gene family analyzed [56] . The phylogenetic tree described above was fitted to CAFE’s requirements by converting it to an ultrametric tree using TreeEdit v1.0, and converting the branch lengths to integers using a custom Python script. The search for λ values was run with the -s option, which specifies an optimization algorithm that finds the values of λ that maximize the log likelihood of the data for all families. For all gene families with significant family-wide P -values, CAFE also runs a Viterbi algorithm that assigns branch-specific P -values for expansions and contractions of each family at each branch of the tree. To infer E. rubrum -specific gains and losses, we used a significance threshold of 0.05 and selected those families with significant Viterbi P -values for E. rubrum , and gains/losses of three or more copies. Microarray design and hybridization The Agilent Technology’s eArray microarray design tool ( https://www.earray.chem.agilent.com ) was used to design up to four 60-mer oligonucleotide probes (total: 39,437 probes) corresponding to protein coding sequences (10,076 CDS in E. rubrum v1.0 release). While most of the CDS received four microarray probes, a few CDS could be assigned only with fewer probes (371, 212 and 12 CDS with three, two or only one probe, respectively). The eArray probe design tool was not able to design microarray probes for nine CDS. Mycelia of Eurotium rubrum (CBS 135680) were grown for 7 days at 27 ° C under different salinity conditions in liquid culture of GY media prepared with 5%, 30%, 50% v/v sterile DSW, an equivalent of brines with 17.4, 104.2 and 173.6 g/l total dissolved salts. Total RNA was isolated from fungal mycelia using the Qiagen RNeasy Plant Mini Kit (Qiagen GmbH) following the manufacturer’s instructions. Gene expression experiments were performed using a custom-made microarray (Agilent Technologies) containing 39,437 probes. Labelled cDNA was prepared from 200 ng of total RNA using the ‘Low Input Quick Amp Labeling Kit’ (no. 5190-2306, Agilent Technologies) and dye-swap experiments were included in the comparative hybridization design ( Fig. 2 ). The hybridization was carried out following the Two-Colour Microarray-Based Gene Expression Analysis protocol (Manual G4140-90050, Agilent Technologies). Microarrays were scanned using Agilent’s scanner and spots were quantified using Agilent’s feature extraction software. An overview about the samples combined for the four independent-microarray hybridizations is depicted in Supplementary Table 11 . Microarray normalization and differential gene expression analysis Visualization of the log-ratio values (Agilent FE software) revealed that the ‘inner’ (25 to 75) quartile boxes of all four two-colour arrays were significantly asymmetric indicating higher overall gene expression rates in cells grown at 30% DSW ( Supplementary Fig. 5 ), although the median of the log-ratio values of the four comparative expression analyses were close to zero and the 5 and 95 percentiles were almost symmetrical. The asymmetry of at least a part of the data points could be due to for example, the significantly higher growth rates of E. rubrum at 30% DSW conditions ( Supplementary Fig. 1 ). For subsequent analyses, the Babelomics 4 suite [26] was used to apply a second normalization step to facilitate differential gene expression detection. The Agilent raw data files were uploaded to the Babelomics 4 analysis suite ( http://babelomics.bioinfo.cipf.es/ ) using the provided Agilent-two-channel upload script and normalized by running the Agilent two-channels normalization script (provided by Babelomics suite, based on the LIMMA package); the settings for the normalization steps were: background correction: ‘normexp’; within arrays normalization: loess (local regression); between arrays normalization: quantiles. The shape of the normalized dataset could be visualized by a second box plot and showed uniform log-ratio distribution within and across the four microarrays ( Supplementary Fig. 5 ). To correct the resulting list of normalized and log-transformed expression ratios for the two dye-swap experimental designs, the sign of two of the four data sets was changed so that all log-transformed expression ratios represent expression changes in relation to the 30% DSW cultures (30% DSW values as the denominators; see Supplementary Table 11 ). The four microarray data sets were assigned to two microarray classes, the low-to-medium comparative experiments (5/30% DSW), and the medium-to-high salt comparative experiments (50/30% DSW), respectively (see Supplementary Table 11 ). Genes differentially expressed in each of the two experimental classes were identified by two independent one-class comparison analyses using Babelomics suite (test: Limma; multiple test correction: false discovery rate; adjusted P -value: 0.05) ( Supplementary Data 2 and 3 ). GO enrichment analyses were performed using the Blast2GO tool [57] . The entire E. rubrum GO annotation available from DOE-JGI was loaded as the reference annotation in Blast2GO and GO enrichment analyses were conducted using Fisher’s exact t -test (one-tailed, P ≤0.05) independently with each of the significantly induced and repressed gene lists. The resulting tables of enriched-GO terms ( Supplementary Data 4 to 7 ) were used to visualize the identified ontologies (biological process, cellular component and molecular function) on GO graphs ( Supplementary Figures 6 to 16 ). Construction of single-member orthologous families A comparative analysis of genome-wide proteome content of E. rubrum was made to nine Trichocomaceae genomes and two halophilic fungi ( Supplementary Table 4 ). Single-member orthologous clusters were constructed by in-house scripts and programs. At the first step, for each pair of genomes, a set of orthologous gene pairs, based on bidirectional best BLAST hits was constructed. In a second step, pairwise orthologs were expanded to construct a single-member orthologous clusters for all genomes, where for each cluster, all pair of genes in the cluster form bidirectional best BLAST pairs for corresponding two genomes. This resulted in 3421 clusters of orthologous genes for 10 Trichocomaceae species. The addition of two phylogenetically distant halophilic decreased the number of such clusters to 1,002. The orthologous clusters were assigned to the species with the higher content of negatively charged residues (D, E) or excess of negatively charged residues over positively charged ones (D+E)−(K+R+H) ( Supplementary Tables 5 and 6 ). Transporter genes Transporter genes were predicted using BLASTP based on best hit homology to transporter sequences (E-value threshold 1e-05, and at least 50% alignment-length coverage), curated at Transporter Classification Database (TCDB) ( http://www.tcdb.org/ ) E-value threshold 1e−05, and at least 50% alignment-length coverage. How to cite this article : Kis-Papo, T. et al . Genomic adaptations of the halophilic Dead Sea filamentous fungus Eurotium rubrum . Nat. Commun. 5:3745 doi: 10.1038/ncomms4745 (2014). Accession codes: E. rubrum Whole Genome Shotgun project has been deposited at DDBJ/EMBL/GenBank under the accession AWRT00000000 . RNAseq data have been deposited in the SRA database under accession codes SRA050508 . The genome and annotation data are also accessible via JGI fungal genome portal MycoCosm [34] at http://jgi.doe.gov/Eurotium . Microarray data have been deposited in the GEO database (/ www.ncbi.nlm.nih.gov/geo/ ) under accession code GSE44180 .